Large mesopelagic fishes biomass and trophic efficiency in the open ocean With a current estimate of ~1,000 million tons, mesopelagic fishes likely dominate the world total fishes biomass. However, recent acoustic observations show that mesopelagic fishes biomass could be significantly larger than the current estimate. Here we combine modelling and a sensitivity analysis of the acoustic observations from the Malaspina 2010 Circumnavigation Expedition to show that the previous estimate needs to be revised to at least one order of magnitude higher. We show that there is a close relationship between the open ocean fishes biomass and primary production, and that the energy transfer efficiency from phytoplankton to mesopelagic fishes in the open ocean is higher than what is typically assumed. Our results indicate that the role of mesopelagic fishes in oceanic ecosystems and global ocean biogeochemical cycles needs to be revised as they may be respiring ~10% of the primary production in deep waters. Mesopelagic fishes—the small fishes living in the ocean’s twilight zone—form one of the most characteristic features of the open ocean: the deep scattering layer at depths between 200 and 1,000 m, visible in the echosounder display of vessels sailing all oceans [1] . Whereas the mesopelagic fish genus Cyclothone sp. is likely the most abundant vertebrate on earth [2] , mesopelagic fishes remain one of the least investigated components of the open-ocean ecosystem, with major gaps in our knowledge of their biology and adaptations, and even major uncertainties about their global biomass. Trawling estimates suggest that the biomass of mesopelagic fishes is ~1,000 million tons [3] , [4] , a number commonly used in assessments of ecosystem function and the biogeochemistry of the global ocean [5] , [6] . However, even for the original estimate it was stated that ‘most of the gear used to obtain the available information obviously underestimate the biomass present’ [3] , and the efficiency of different types of nets to capture mesopelagic organisms has been further questioned recently, with inter-calibration exercises showing order-of-magnitude differences in the captured biomass depending on the type of gear [7] . Moreover, trawling-based biomass estimates are systematically below acoustic estimates [7] , [8] , [9] , as mesopelagic fishes have been shown to exhibit escape reactions to nets, rendering trawling data suspect of gross underestimation [10] . Here we combine a sensitivity analysis of acoustic data collected during Malaspina 2010, the Spanish Circumnavigation Expedition (December 2010–July 2011, Fig. 1a ), and modelling, to show that mesopelagic fishes biomass in the open ocean is about one order of magnitude higher than previous estimates. We furthermore examine the mesopelagic fishes biomass relative to primary production (PP) and consider the implications of these estimates for the functioning of the open-ocean ecosystem and biogeochemical cycles. 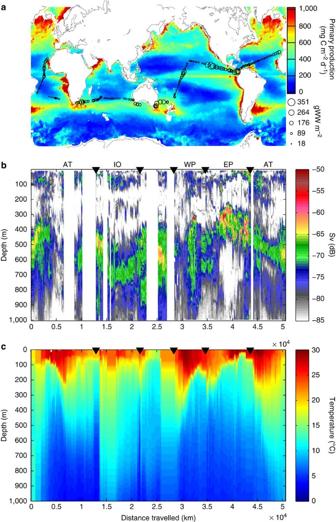Figure 1: The Malaspina cruise. (a) The surface-integrated estimated mesopelagic fishes biomass (g wet weight per m2) for the 200–1,000 m depth range along the Malaspina 2010 Expedition cruise transect (black circles) superimposed on a satellite-derived global map of PP (average in mg C m−2d−1for 2010–colour bar); (b) a daytime echogram from 0–1,000 m along the cruise track (measured in dB—colour bar), and (c) interpolated temperature profiles along the cruise track (measured in °C—colour bar). The black triangles inbandcindicate the border between oceanic basins. AT for Atlantic Ocean, IO for Indian Ocean, WP for Western Pacific and EP for Eastern Pacific. Figure 1: The Malaspina cruise. ( a ) The surface-integrated estimated mesopelagic fishes biomass (g wet weight per m 2 ) for the 200–1,000 m depth range along the Malaspina 2010 Expedition cruise transect (black circles) superimposed on a satellite-derived global map of PP (average in mg C m −2 d −1 for 2010–colour bar); ( b ) a daytime echogram from 0–1,000 m along the cruise track (measured in dB—colour bar), and ( c ) interpolated temperature profiles along the cruise track (measured in °C—colour bar). The black triangles in b and c indicate the border between oceanic basins. AT for Atlantic Ocean, IO for Indian Ocean, WP for Western Pacific and EP for Eastern Pacific. Full size image Acoustic biomass estimates A Simrad EK60 echosounder operating at 38 kHz frequency was used to obtain data throughout the 32,000-mile voyage ( Fig. 1a ). We used data obtained during the daytime from 200–1,000 m depths, comprising the main diurnal habitat of mesopelagic fishes, to calculate fish biomass and considering the different sources of uncertainties involved (Methods). The average (±s.d.) nautical area scattering coefficient ( s A , m 2 nmi −2 ) in the 200–1,000 m layer for the whole cruise was 1,864±1,341, with individual estimates ranging from 158–7,617 m 2 n mi −2 ( N =209, Fig. 1a,b ). The s A was significantly correlated with the 2010 satellite-derived average daily PP (mg C m −2 d −1 ) [11] , ( Fig. 2 , Pearson’s r =0.77, F corrected for spatial autocorrelation=26, D.F. corrected for spatial autocorrelation=18, P <0.01). This relation shows heteroscedasticity ( Supplementary Fig. 1 ) and because of the cruise design (from coast to coast at similar distances) it also shows spatial autocorrelation at different spatial scales (Moran I test, Supplementary Fig. 2 ) [12] . Therefore, we used a geographically weighted regression (GWR) [13] on ln-transformed values to parameterize the relationships between PP and s A through regression analysis (Methods). The GWR was significant in 96% of the sampling points, ranging from oceanic gyres to near shelf areas ( Supplementary Fig. 3 ). The only area where the GWR was not significant was in the vicinity of the Humboldt upwelling system where the water column was severely hypoxic below 100 m ( Supplementary Fig. 4 ). 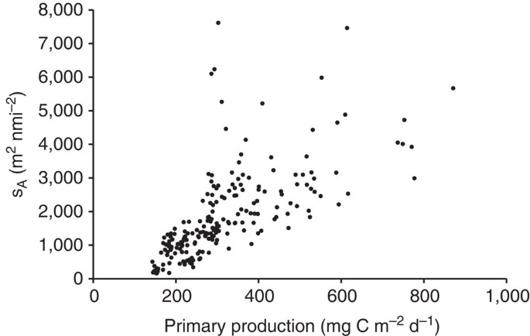Figure 2: Relationship between PP and acoustic backscatter. The relationship between PP (2010 annual average mg C m−2d−1) and the nautical area scattering coefficient (sA, m2nmi−2) from 200–1,000 m during day time. Figure 2: Relationship between PP and acoustic backscatter. The relationship between PP (2010 annual average mg C m −2 d −1 ) and the nautical area scattering coefficient ( s A , m 2 nmi −2 ) from 200–1,000 m during day time. Full size image We used the equations obtained through the GWR in two ways to derive estimates of the s A from satellite-estimated PP: first, the median values of all the GWR parameters and second, as the regression parameters above 400 mg C m −2 d −1 of PP show less variability ( Supplementary Fig. 5 ), we also considered different equations with the median values for data below and above 400 mg C m −2 d −1 ( Supplementary Table 1 ). Use of the relation between PP and s A ( Fig. 2 ), together with the distribution of PP, to integrate mesopelagic fishes biomass for areas with bottom depths deeper than 1,000 m between 40° N and 40° S (the latitudinal range covered by the Malaspina expedition, Fig. 1a ) yielded a total s A of 5.6 × 10 17 ( Table 1 ). Table 1 Acoustic fishes biomass estimates. Full size table We transformed the backscattering strength integrated over the 200–1,000 m layer, s A , into mesopelagic fishes biomass using db/weight ratios derived from the literature ( Table 2 ). To account for the variability in these ratios we considered the minimum, maximum, average, median, 25 and 75% quartiles of the literature values. Table 1 presents the range of mesopelagic fishes biomass obtained using different approaches to estimate the total s A between 40° N and 40° S (ordinary least squares regression, GWR, average s A from the cruise) and db/weight ratios. We found that total mesopelagic fishes biomass was robust against different approaches to estimate s A with a difference of 25% between the maximum (GWR) and the minimum (cruise average). If we consider the range between 25 and 75% quartiles of the literature db/weight ratios as a reasonable representation of the mesopelagic fishes around the world, our estimates of mesopelagic fishes biomass would range from 6,000–200,000 million tons, with median values between 11,000 and 15,000 million tons ( Table 1 ). These estimates of mesopelagic fishes biomass limited to 40° N and 40° S are one order of magnitude higher than the previous global estimate of 1,000 million tons [3] , [4] . Table 2 Target strength of mesopelagic fishes at survey frequencies. Full size table As mesopelagic fishes are not the only source of backscatter we conducted a sensitivity analysis to understand which combinations of db/weight ratios and fraction of the backscatter coming from fishes would result in the present day estimate of 1,000 million tons. 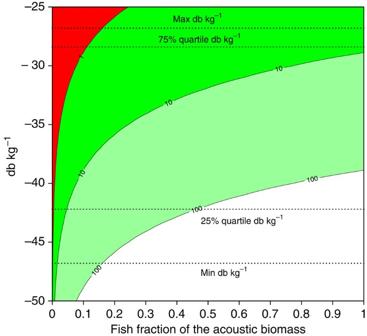Figure 3: Sensitivity analysis of the assumptions used to estimate biomass. Computations are based on the total backscatter estimated from the GWR regression (Table 1, 5.57E+17), contours are the ratio of our estimate to 1,000 million tons. Quartiles, maximum and minimum values of the db/weight ratios found in literature are indicated by the dotted lines. Figure 3 shows that the present day estimate can only be attained if all mesopelagic fishes populations had a db/weight ratio close to the maximum observed in the literature and mesopelagic fishes represented <20% of backscatter or if they were <10% of the backscatter for a wider distribution of db/weight values ( Fig. 3 ). Any contribution to the backscatter higher than 20%, as generally reported [9] , [14] , results in a biomass several times higher than the one accepted ( Fig. 3 ). Figure 3: Sensitivity analysis of the assumptions used to estimate biomass. Computations are based on the total backscatter estimated from the GWR regression ( Table 1 , 5.57E+17), contours are the ratio of our estimate to 1,000 million tons. Quartiles, maximum and minimum values of the db/weight ratios found in literature are indicated by the dotted lines. Full size image Modelling biomass estimates Global fishes biomass estimates derived from food web models are typically between 900 and 2,000 million tons [15] , [16] , [17] , about 10-fold below our direct, acoustic measurement. In some of those models, the mesopelagic biomass is an input affecting total fishes biomass estimates [15] ; in others the final value is very sensitive to the transfer efficiency used [16] , and finally, the most recent work by Tremblay-Boyer et al. [17] using ECOTROPH [18] derived its estimate of fishes biomass assuming that 10% of the PP was transferred from PP to herbivores (Gascuel pers. comm.). This value of 10% corresponds to the consumption of PP by mesozooplankton in productive areas (mainly copepods) [19] . Yet, ample evidence shows that microzooplankton, not mesozooplankton, are the major consumers of PP, consuming 70–80% of the PP on average [20] . The percentage of the PP consumed by mesozooplankton in the less productive oceanic waters is also more likely to be ~20% rather than 10% (ref. 19 ). Therefore, if we consider micro and mesozooplankton together the percentage of PP entering the food web should be closer to 90%. Hence, we have run the ECOTROPH model with a generic open-ocean ecosystem model using the average PP for the area between 40° N and 40° S (344 mg C m −2 d −1 ) and considering a flux from PP to the trophic web of 70, 80 and 90%, with transfer efficiencies between trophic levels ranging from 0.05 to 0.2 (ref. 21) [21] and an average temperature of 9 °C. Results, shown in Table 3 , range from 2,000–70,000 million tones. Table 3 Fishes biomass Ecotroph estimates. Full size table Both along the Malaspina transect ( Fig. 4 ) and in the global estimate ( Table 3 ), the modelled biomasses using ECOTROPH with a transfer efficiency of 10% fall within the range of acoustic estimates using the median db/weight ratio (10–15,000 million tons). 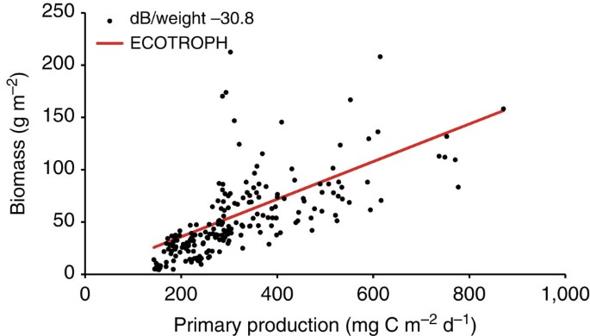Figure 4: Relation between PP and fish biomass. The relationship between PP (2010 annual average mg C m−2d−1) and the estimated mesopelagic fishes biomass using the median db/weight ratio (black circles) and the ECOTROPH model with a transfer efficiency of 0.1 and considering that 90% of the PP enters the food web (red line). The regression equation of the acoustic biomass estimate against PP is mesopelagic fishes biomass (g m−2)=0.185 PP (mg C m−2d−1)—6.66,r2=0.46,P<0,001,n=209). Figure 4: Relation between PP and fish biomass. The relationship between PP (2010 annual average mg C m −2 d −1 ) and the estimated mesopelagic fishes biomass using the median db/weight ratio (black circles) and the ECOTROPH model with a transfer efficiency of 0.1 and considering that 90% of the PP enters the food web (red line). The regression equation of the acoustic biomass estimate against PP is mesopelagic fishes biomass (g m −2 )=0.185 PP (mg C m −2 d −1 )—6.66, r 2 =0.46, P <0,001, n =209). Full size image Production and transfer efficiency We estimated mesopelagic fishes production (MFP) considering equations relating fishes production/biomass (P/B) ratios to the trophic level, assumed to be 3.2 for mesopelagic fishes ( www.Fishbase.org ) and temperature [22] , which was derived from temperature profiles weighted by the depth distribution of the fishes biomass ( Fig. 1b,c ). This resulted in an average P/B for mesopelagic fishes of 0.5 (average±s.d. 0.51±0.05). Biomass was estimated in a conservative way using the median and 75% quartile of the literature db/weight ratios. As the mean-weighted temperature in the deep layers was relatively uniform (average 9 °C, range 6 °C to 13 °C, Fig. 1c ), we found that MFP was also significantly correlated to PP (Pearson’s r =0.68, F corrected for spatial autocorrelation=21, D.F. corrected for spatial autocorrelation=26, P <0.01). The average MFP values calculated along the Malaspina 2010 transect ranged between 16 and 27 g m −2 y −1 (average±s.d. MFP=27.2±20.1 and 15.6±11.6 g m −2 y −1 for median and 75% quartile db/weight ratios). The corresponding average transfer efficiency from PP (TL1) to MFP (TL3) was 0.02 (average±s.d. MFP/PP ratio=0.022±0.013) when using the median db/weight ratio and 0.01 when using the 75% quartile (average±s.d. MFP/PP ratio=0.013±0.008) ( Fig. 5 ). 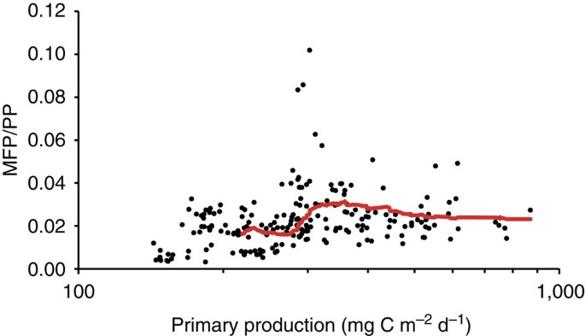Figure 5: Trophic efficiency. The estimated trophic efficiency from PP to MFP (the ratio of fishes production to PP) as a function of PP. The line is a 50 period running average for 50 contiguous estimates. Figure 5: Trophic efficiency. The estimated trophic efficiency from PP to MFP (the ratio of fishes production to PP) as a function of PP. The line is a 50 period running average for 50 contiguous estimates. Full size image Through the use of acoustic data deeper than 200 m and considering the open-ocean areas between 40° N and 40° S with bottom depth deeper than 1,000 m and trophic levels 3–3.5 this analysis focuses on mesopelagic fishes, excluding fishes living in shelf areas, epipelagic fishes and higher-level predator fishes in the open ocean. Our results indicate that the mesopelagic fishes biomass in the global ocean is much higher than the previous estimate of 1,000 million tons [3] , [4] . The sensitivity analysis ( Fig. 3 ) indicates that a better knowledge of the composition and acoustic properties of the mesopelagic community is needed to obtain accurate estimates of the biomass. However, considering the agreement between the acoustic estimate using the median db/weight value and the model using 10% efficiency between trophic levels we suggest that the most likely estimate of mesopelagic fishes biomass between 40° N and 40° S is at least an order of magnitude higher than the previous estimate of 1,000 million tons. Our analysis is limited to the latitudinal range covered by the Malaspina expedition (40° N–40° S). Yet, mesopelagic fish are also abundant in higher latitudes, although their abundance strongly decreases in polar waters. Considering only the surface of the area the estimate could be ~30% higher if expanded to the deep ocean between 70° N and 70° S. Actually, the biomass levels we find using acoustics and the median db/weight, as well as the relation between PP and mesopelagic fishes biomass, agree well with recent observations in the northeast Pacific Ocean [23] . Both our estimate using acoustics and the local estimates in the northeast Pacific Ocean coincide in biomasses one order of magnitude higher than previous estimates. As mesopelagic fishes likely dominate the global fishes biomass even with the former estimate, our results indicate that the current global fishes biomass needs to be upgraded by one order of magnitude. Primary production in the oligotrophic ocean is dominated by picoplankton [24] , which are not efficiently captured by copepods. It is therefore generally implied that the ‘microbial loop’ dominates the trophic web in oligotrophic areas, which therefore should support a lower transfer efficiency from PP to mesozooplankton, and hence to fishes, than more productive marine systems [25] . However, there is no direct evidence of a lower efficiency in less productive areas [26] . On the contrary some data suggest a tighter coupling between PP and grazing in oligotrophic seas [19] . Although a transfer efficiency of 0.1 between consecutive trophic levels is commonly assumed, values of 0.2 and higher are also used in trophic models of aquatic ecosystems [21] . Recent studies have shown that food-transfer efficiencies can vary several orders of magnitude, from less than 0.001 to significantly more than 0.1 (ref. 27 ). The transfer efficiency between consecutive trophic levels implicit in our transfer efficiency estimates between TL1 and TL3 appears to be in conflict with the common wisdom that trophic chains in oligotrophic systems are less efficient than in productive shelf waters [28] (generally considered to be 0.1). However, the transfer efficiency from PP to microzooplankton is probably higher in warm areas of the ocean (oligotrophic zones) than in eutrophic areas, as grazing by heterotrophs is more tightly coupled to PP in warmer seas where heterotrophic metabolic rates increase faster than phototrophic rates relative to increases in temperature [29] . Further, the dominance of pico-sized primary producers in the oligotrophic ocean [24] implies small losses due to sinking particles. Mesopelagic fishes are visual predators feeding on mesozooplankton (TL3–4, see Methods). The trophic transfer efficiency from mesozooplankton to fishes is also probably higher in less productive and clear oceanic waters than in more productive and turbid shelf and coastal waters ( Supplementary Table 2 ): clear water has a low beam attenuation coefficient ( c ), which affords visual predators long sighting distances ( r ), according to r = k / c , where k is determined by the contrast and the contrast sensitivity of the prey and the predator, respectively [30] . The volume searched per unit time ( V ) scales with r 2 for a cruising predator [31] and is therefore effectively enhanced by decreased c (that is, increased water clarity) according to V ∝ c −2 (Methods). In addition, clear water also has a low attenuation coefficient for downwelling irradiance ( K ), which means that light penetrates deeper. Within the range allowed by deep hypoxic layers [32] , evidence suggests that vertical extension of fishes habitat ( H ) scales according to H ∝ 1/ K (ref. 33 ). Thus, increased water clarity tends to increase both the short ( r ) and the long ( H ) range for visual foraging, thereby enhancing the transfer efficiency from mesozooplankton to mesopelagic fishes through more effective visual predation. The quantity c −2 K −1 , which is proportional to the potential volume searched, is about one order of magnitude higher for clear oceanic water ( K =0.044 m −1 , the average in our study) than for turbid coastal waters with K >0.1 m −1 ( Supplementary Table 2 ). Thus, although increased PP in productive areas is likely to increase production at TL2 and TL3, it is also likely, beyond a certain point where high plankton biomass leads to high light attenuation and visual constraints become severe, to decrease the transfer efficiency between mesozooplankton and visual predators [34] relative to the transfer efficiency in clear waters at the oligotrophic ocean. The evidence that mesopelagic fishes biomass, and consequently the total fishes biomass, is 10-fold higher, or even more, than previously assumed has important implications for our understanding of the carbon fluxes in the ocean. A discrepancy in the estimates of export production using 234 Th: 238 U disequilibria and shallow sediment traps has been systematically reported [35] . This discrepancy has generally been attributed to artifacts in the traps [36] or to the episodic nature of the sinking events [37] . A comparison between reverse modelling estimated C export fluxes and sediment traps suggested that shallow traps (<1,000 m) underestimate the flux, whereas deep traps (>1,000 m) measured fluxes higher than the modelled ones [38] . An order of magnitude higher biomass of mesopelagic fishes might explain the difference. Mesopelagic fishes perform diel vertical migration, feeding at night in the upper layers (euphotic) and excreting and respiring at depth at day. This implies that mesopelagic fishes drive a vertical flux from the surface to the mesopelagic layer, bypassing the detection capacity of sediment traps. At the same time, by defaecating in deep waters, faeces produced with surface organic matter start sinking at depths of ~500–700 m, bypassing consumption in a large fraction of the water column and increasing the observed flux in deep traps. Basically, mesopelagic fishes accelerate the flux by actively transporting organic matter in the top layer of the water column, where most organic carbon is lost from the sedimentary particle flux. Del Giorgio and Duarte [39] , using fishes production estimates derived from fisheries landings (mesopelagic fishes are not commercially fished), considered fishes respiration of little significance for the global ocean. However, a substantial revision of the mesopelagic fishes biomass upwards renders fishes respiration relevant. Assuming fishes respiration to be nine times production [39] and half of it to happen in deep waters, up to 10% of the PP could be respired by mesopelagic fishes in deep waters ( Table 4 ). This estimate is again in agreement with the local estimate in the northeast Pacific [23] . The estimate needs refinement in terms of time occupied and the respiration rates in deep layers (usually more than half of the day, but also at low temperatures), but indicates that, in deep layers, the sum of MFP and respiration is in the order of magnitude needed to explain the discrepancies between 234 Th: 238 U disequilibria and shallow sediment traps. Moreover, the excretion in deep layers of materials ingested by mesopelagic fishes in the surface might partly explain the unexpectedly large microbial respiration in the deep ocean [40] . Table 4 Fish production and respiration estimates. PP, MFP and respiration estimates along the Malaspina transect. Full size table Our results strengthen the previous claim that mesopelagic fishes are the most abundant fishes and, indeed, the most abundant vertebrates in the biosphere [2] . The results from the survey presented here suggest that trophic transfer efficiency from primary producers to fishes has been underestimated in the oligotrophic ocean, with the high transfer efficiency from primary producers to fishes associated with warm water temperatures and extreme water transparency, maximizing prey capture by visual predators. As many mesopelagic fishes, dominant in oceanic areas, are strong vertical migrators, feeding in the upper water column and excreting at depth, these results have important implications for the biogeochemical cycles of the ocean, as these animals provide trophic connectivity and transport organic carbon between the surface and the mesopelagic ocean, and could help explain existing discrepancies between flux estimates obtained by the 234 Th: 238 U method and sediment traps [35] , as well as the unexpectedly large microbial respiration in deep water [40] . Even with the current 10 9 tons estimate mesopelagic fishes are considered to play a key role in the world’s oceans as a link between plankton and top predators [41] and in the oxygen depletion of the open ocean deep layers [32] . With the 10-fold higher biomass found in this study and in recent local studies [23] the conclusion about potential impacts of harvesting mesopelagic fishes extends to the global biogeochemical cycles. This finding calls for an effort to improve the accuracy of the estimates of the biomass and composition of the mesopelagic community. A more accurate estimate will require technological developments to increase the capturability of mesopelagic fishes and obtain detailed target strengths, as well as coordinated cruises across representative areas of the world ocean with sufficient resolution to address mesoscale structures. Echosounder Continuous acoustic measurements were made with a calibrated [42] Simrad EK60 echosounder (7° beam width), operating at a frequency of 38 kHz and with a ping rate of 1 transmitted pulse per 2 s. The data were stored for later analysis, carried out using the LSSS software [43] . The echosounder data were episodically affected by noise from various sources; consequently, prior to import into the LSSS software for post-processing, the data were subjected to a series of filters to remove bad data. These filters introduced a bias by removing the highest intensity data, however. The backscatter estimates, which are the basis of our biomass estimates, are therefore conservative. The filters worked by comparing the integrated backscatter over a depth range with the background backscatter over the same depth range. Background intensities were detected using a median filter that was 400 pings wide, updated every 100 pings. Pings affected by attenuation were defined as pings with backscatter >6 dB below the median in either of the depth ranges of 50–600 m or 600–1,000 m. Periods with backscatter >4 dB above background levels in the depth range 800–1,000 m were also marked. Pings tagged by these filters were excluded in further analyses. Lastly, a simple 9-point running median (horizontal) removed shorter irregular spikes. After manual scrutiny of the remaining data, the data were integrated in 2-minute-by-2-metre bins at a threshold of −90 dB. After integration in LSSS, data were imported into R [44] for further analysis. Acoustic results were split into day, night and crepuscular data, using the function ‘sunriset’ from the ‘maptools’ package, with crepuscular periods defined as sunset/sunrise±1 h. To plot the echogram ( Fig. 1b ), the processed LSSS data were exported in 10-minute-by-1-metre bins to Matlab, where the nautical area scattering coefficient ( s A , m 2 nmi −2 ) was converted to volume backscattering strength ( S v , dB re 1 m −1 ). The daytime data were extracted (2 h after sunrise and 2 h before sunset) and interpolated to remove the night-time gaps. Longer distances with missing or removed data (between cruise legs) were plotted as white. Satellite data The satellite data we used were all annual averages for the year 2010. Annual averages of PP for 2010 were generated by averaging monthly data for PP downloaded from the Ocean Productivity website ( http://www.science.oregonstate.edu/ocean.productivity/index.php ) [11] . Cruise segments were then generated by combining all position fixes within a startpoint±(8 × 4.6) km in north, south, east and west directions. The startpoint of the next segment was the first position registered outside this box. Alignment of in situ and satellite data was done by selecting the 64 (8 × 8, size per bin ~4.6 × 4.6 km) chlorophyll- a bins along the segments that were closest to the midpoint (median position) within a cruise segment, with the added restriction that no chlorophyll- a bin could be used twice. Values for these 64 bins, corresponding to an area of ~37 × 37 km were averaged. For the other satellite-derived measurements, the maximum and minimum positions of the chlorophyll- a bins were used as boundaries for selection prior to calculation of the averages. Data from the conductivity temperature and depth (CTD) probe were aligned to cruise segments, and only CTD casts within a given cruise segment were used for a given segment. Areas for biomass estimation We used the PP–backscatter relation to estimate the mesopelagic biomass from satellite-derived PP data. We determined the biomass from the sum of the biomasses estimated from satellite-derived PP estimates using only areas where the bottom depth was >1,000 m. We used the ETOPO1 data set ( http://www.ngdc.noaa.gov/mgg/global/global.html ) to estimate the area. The bathymetry data set was translated down to a 10′ arc grid, and for every cell in the PP data set grid (~same spatial resolution, not identical grids), we assigned the depth from the closest grid-point in the bathymetry data set. Primary production grid-points/cells with bottom depths shallower than 1,000 m were then excluded from our biomass estimation, as were areas north and south of 40 degrees north and south. This resulted in an area of 222.3 million km 2 . Temperature data The temperature data to estimate the MFP/biomass ratio (P/B) were obtained from the Malaspina Expedition CTD profiles. Profiles inside the PP boxes, or those closest to the boxes were used. As more data-points were available for daytime, we used the temperature at the daytime weighted mean depth (WMD) of the acoustic data. In areas where day- and night-time acoustic WMDs were available, the average difference between the daytime WMD temperature and the average temperature between day- and night-time WMD was <0.1 °C (see Supplementary Table 3 ). Modelling The model ECOTROPH [18] was run using the plugin incorporated to Ecopath with Ecosim [45] , (EwE, www.Ecopath.org ) and the generic model Ocean Ecost as a basis. We used the average PP for the oceanic area deeper than 1,000 m between 40°N and 40°S (344 mg C m −2 d −1 , http://www.science.oregonstate.edu/ocean.productivity/index.php ), considering a flux from PP to the trophic web of 70, 80 and 90% (ref. 20 ), transfer efficiencies between trophic levels ranging from 0.05 to 0.2 (ref. 21) [21] and a temperature of 9 °C (see above). ECOTROPH estimates biomass and production per trophic level (TL) in steps of 0.1 and we considered mesopelagic fishes as the main community between TL 3 and 3.5 in the open sea and biomass estimates are provided for that range. Mesopelagic fishes generally feed on zooplankton organisms such as copepods and euphausiids ( www.fishbase.org ). To determine the TL of mesopelagic fishes we used fishbase ( www.fishbase.org ) with searches for ‘lanternfish’ and ‘bristlemouths’ (myctophids and Cyclothone sp.). This yielded 96 and 15 TL values for lanternfish and bristelmouths respectively. For lanternfish the TL ranged from 3 to 4.6, with an average of 3.2, mode of 3.1 and median of 3.2. For bristelmouths the TL ranged from 3 to 3.6, with an average of 3.3, mode of 3.5 and median of 3.3. Biomass transformations For comparison, fishes production and PP were transformed from carbon into wet weight using a factor of 10:1 (ref. 21 ). Statistics Area scattering coefficient ( s A ) was significantly correlated to PP. However, straight regression between the two factors ( s A =2374 ln (PP)+11624) was limited by the heteroscedasticity of the data ( Supplementary Fig. 1A ). In principle heteroscedasticity does not affect ordinary least squares regression coefficient estimates, but can bias the significance estimates. Logarithmic transformation of the data (ln ( s A )=1.52 ln (PP)–1.36) eliminates heteroscedasticity ( Supplementary Fig. 1B ) but still presents spatial autocorrelation ( Supplementary Fig. 2 ), that can increase type I errors [12] . GWR is a method to obtain regression parameters for each of the points in a spatial grid using the surrounding points weighted by distance. In spatial analysis GWR offers the advantage of extracting additional information at each location, as well as usually not being affected by spatial autocorrelation [13] . Here we carried a GWR regression on ln-transformed data using a bi-square spatial weighting function and a bandwidth of 4,130 units. The regression was performed using the Spatial Analysis in Macroecology software (SAM), [46] . Supplementary Table 1 presents the comparison of the three regressions in terms of parameters estimates, r 2 and Akaike coefficient. Supplementary Fig. 3 presents the spatial variations of the significance of the GWR slopes. The slopes were generally highly significant except in the Eastern Pacific, near the Humboldt current, where the layers below 100 m showed severe hypoxia ( Supplementary Fig. 4 ). This suggests that the s A –PP relation is affected in that specific area either because severe hypoxic conditions influence the niche space, or because there is a strong external input of organic matter and local PP does not reflect the food conditions. Regardless, the type of regression used to estimate s A from satellite PP has a limited effect on the overall biomass estimate (see Table 1 ). The K- and c-effects on vision-based feeding habitats Both the beam attenuation coefficient ( c , m −1 ) and the downwelling irradiance attenuation coefficient ( K , m −1 ) are affected by water clarity. We compared the quantity c −1 K −2 , which is proportional to a theoretical search volume, for clear oceanic and less clear coastal water ( Supplementary Table 2 ). The quantity c −1 K −2 has unit m 3 and combines the effects that water clarity has on the short ( r , the sighting distance) and the long ( H , the vertical extension of the habitat) range search ability of a vertically migrating visual predator. The sighting distance is [30] : where k =ln( C 0 / C min ), C 0 is the inherent contrast of the prey, and C min is the minimum contrast that the predator can detect [30] . The vision-based prey detection rate ( p ) for a cruising predator tends to be proportional to r 2 (ref. 47 ), which in combination with Equation (1) gives: A fish that migrates vertically has a larger potential feeding habitat than a fish that remains at the same depth. A greater area of migration also provides a larger potential feeding habitat [48] . Within the range allowed by oxygen levels [32] , for a fish with a certain light preference (isolume), the migration distance ( H , m) scales with K according to refs 33 , 47 : The product of the right-hand side of Equations (1) and (2), c −2 K −1 (m 3 ), combines the optical characteristics of the short- and the long-range search ability of a vertically migrating predator. We approximated this quantity, which is proportional to a theoretical search volume, for the average water clarity of the stations of the cruise and for hypothetical coastal waters with K -values of 0.10 and 0.15, which are in the lower range of those reported in Table 6.2 in the study by Kirk and Light [49] . According to Supplementary Table 3 , the estimate of this search volume is about one order of magnitude higher for the average Malaspina station than for the hypothetical coastal waters. This suggests that, in order for the vision-based prey detection rates to be equal, the prey concentration must be 10 times higher at the coastal location, assuming all other factors to be equal. This suggests that the high clarity of oceanic water enables efficient visual feeding at low prey concentrations. Uncertainty analysis Transforming acoustic measures into biomass involves uncertainty, dependent on the distribution of fishes sizes relative to acoustic wave lengths, on correctly ascribing the acoustic backscatter to fishes in scattering layers composed of different taxonomic groups as well as on the use of appropriate conversion factors from backscatter to biomass (TS values). In order to assess the bias introduced through our non-standard post-processing methods, we compared our results with results from standard acoustic post-processing in selected low-noise sections. Standard post-processing here refers to automated removal of noise spikes and background noise as implemented in the software LSSS, in addition to manual scrutiny of data and removal of periods where these automated filters did not eliminate all noise, or removed substantial portions of the data. Results are presented in Supplementary Figs 5 and 6 as a fraction of the difference between standard results and our results (only 200–800 m data, standard s A –filtered s A /filtered s A ). Fractions were averaged either per depth channel ( Supplementary Fig. 6 ) or per time bin ( Supplementary Fig. 7 ). Time-averaged results ( Supplementary Fig. 7 ) suggest that there is a linear relationship between our estimates and standard estimates, with our estimates ~30–40% lower than standard estimates. The vertical bias profile ( Supplementary Fig. 6 ) shows that there is a vertical influence on the bias, but that the bias appears almost constant at 30–40% in the 400–800 metre depth range (suggesting the magnitude of underestimation for this depth range, encompassing most of the mesopelagic backscatter; cf . Supplementary Fig. 6 ). The bias is higher at depths shallower than 400 m; it drops rapidly at depths lower than 800 m, suggesting that there is no bias at ~900 m and a negative bias deeper than this (that is, our estimates are higher than standard estimates at these depths). The taxonomic composition of the organisms responsible for the mesopelagic backscatter along the path of this circumnavigation voyage is not known. Moreover, not all of the backscatter originates from fish. Early studies of the deep scattering layer concluded that larger crustaceans and in particular euphausiids were significant in the deep scattering layer [50] , but later studies showed that at the low frequencies used in these early studies, mesopelagic fish were the most significant scatterers, although with a possible contribution from gas-bearing siphonophores [51] . Larger crustaceans are relatively weak scatterers compared with organisms with air-inclusions at the frequency used in this study [52] , and therefore they probably made up a negligible proportion of the total backscatter at our frequency. Accordingly, recent studies from oceans around the world conclude that mesopelagic fish make up the majority of the backscatter [9] , [14] yet proper ‘ground truthing’ is not possible due to the highly varying catch efficiency of sampling gear [7] , which renders estimates derived from nets unreliable. Size of the fish is another potential issue. At 38 kHz the acoustic wave length is ~3.9 cm. Individuals much smaller than the wavelength can be detected, particularly when occurring in high concentrations (although mesopelagic fish do not school). There is, however, an exponential decrease in acoustic backscatter with decreasing size in this so-called Rayleigh scattering region [53] . It is likely that a large part of the mesopelagic fish community is smaller than 3.9 cm. This would lead to underestimating mesopelagic fish biomass, as fish in the Rayleigh domain would result in small db/weight ratios, except for individuals with a resonant swim bladder. Resonance has the potential to result in a large bias of the estimate by directly affecting the acoustic results by up to 25 times [54] . Swimbladder resonance may increase acoustic backscatter from small mesopelagic fish and organisms with air bubbles [55] . However, although a certain level of resonance cannot be excluded, the data suggest that is not a major source of bias because (1) the ratio of paired day and night backscatter values is generally <1, (2) if resonance was high and widespread the geographically weighted relation between s A and PP should disappear and (3) the ecotroph model results agree well with the acoustic estimate. Modelling and field studies suggest that the effects of resonance at 38 kHz increase with depth [9] , [56] . Therefore, if the resonance effect was a major bias in our data set, we would expect the total night-time backscatter to be much lower than corresponding daytime values, because, on average, animals are distributed considerably closer to the surface at night, and thus producing lower resonance. We would also expect to observe high variability in the day/night ratio along the transect when going over different communities (fish species and sizes) with different resonance levels. We therefore compared day and night column (10–1,000 m) total backscatter values to check for the potential influence of resonance in our data. The ratio of paired day and night backscatter values ( Supplementary Fig. 8 day s A /night s A ) shows that most of these values are <1 with low variability (average day/night ratio value 0.96, s.d. 0.53). The vertical bias would tend to drive this ratio in the same direction as resonance, while migrations from deeper in the water column would oppose the trend. Our low ratios are inconsistent with resonance being a major factor. However, in one section along the cruise-track (East Pacific), the ratios appear to be higher (2–3), consistent with resonance playing a role. This is the same zone, with hypoxic waters at 100 m (see Supplementary Fig. 4 ), where the GWR is not significant. However, the biomass estimates in that area are not outliers in the general regression ( Supplementary Fig. 9 ) or higher than that predicted by Ecotroph for the zone ( Supplementary Fig. 10 ), which suggests that the day/night ratios >1 could be explained by factors other than an overestimation of the biomass. In this region, the night-time vertical profiles were particularly close to the surface, suggesting that a large proportion of the biomass actually migrates to the near-surface dead-zone of the echosounder, leading to a lower total night-time backscatter [57] . In any case the data from that limited area do not influence the estimations of global backscatter using different methods (regressions or average). The spatial coherence of the GWR (GWR parameters and significance) is also a strong indication that resonance does not play a major role. Unless resonance was the same all along the transect (same community composition, sizes, depth distribution and migration patterns all around the world), resonance should eclipse the local relation between s A and PP in areas where resonance was relevant. The GWR does not show such variability and the relation remains significant all along the transect, except for the North East Pacific area with hypoxic deep layers that also show higher day/night ratios ( Supplementary Fig. 4 ). Finally, the general estimate and the estimations along the transect agree with the Ecotroph model results using average parameters. The model is completely independent from acoustics estimates, based on PP and transfer efficiency. The agreement between the two independent approaches suggests that resonance is not a major source of bias in the acoustic data. We use a range of literature db/weight ratio values to estimate biomass. This is a simplification that precludes exact estimation at each single point, but is largely to generate reliable average estimates, as the inaccuracies go both ways. A large portion of the backscatter from an individual fish normally originates from its gas-filled swimbladder [52] , but in mesopelagic fish reduced swimbladders or fat-filled swimbladders are common [58] and have a strong effect on the TS of the fish. For instance, adults of some species of the genus Cyclothone may have gas-filled swimbladders, whereas only juveniles in other Cyclothone species have gas-filled swimbladders. There are other species of the same genus that never have gas-filled swimbladders [58] . Ground truthing in each area is not possible, but the 25–75% quartile range used in the estimates provided here should encompass the average TS value for the oceanic mesopelagic fish populations. As our focus was mesopelagic fish, we did not include the backscatter from the upper 200 m layer (apart from the test on resonance). The additional fish biomass in the upper 200 m would contribute to a higher biomass estimate of total fish. The integrated s A for the upper layer is on average 27% of the integrated value from 200–1,000 m. However, if five areas with exceptionally high values were excluded, the average value would drop to 7% ( Supplementary Fig. 11 ). How to cite this article: Irigoien, X. et al. Large mesopelagic fishes biomass and trophic efficiency in the open ocean. Nat. Commun. 5:3271 doi: 10.1038/ncomms4271 (2014).